Sensitive magnetic control of ensemble nuclear spin hyperpolarization in diamond Dynamic nuclear polarization, which transfers the spin polarization of electrons to nuclei, is routinely applied to enhance the sensitivity of nuclear magnetic resonance. This method is particularly useful when spin hyperpolarization can be produced and controlled optically or electrically. Here we show complete polarization of nuclei located near optically polarized nitrogen-vacancy centres in diamond. Close to the ground-state level anti-crossing condition of the nitrogen-vacancy electron spins, 13 C nuclei in the first shell are polarized in a pattern that depends sensitively upon the magnetic field. Based on the anisotropy of the hyperfine coupling and of the optical polarization mechanism, we predict and observe a reversal of the nuclear spin polarization with only a few millitesla change in the magnetic field. This method of magnetic control of high nuclear polarization at room temperature can be applied in sensitivity enhanced nuclear magnetic resonance of bulk nuclei, nuclear-based spintronics, and quantum computation in diamond. Several techniques based on spin polarization transfer have been developed to enhance the magnetization of nuclei. They are applied widely in NMR-based probes of the chemistry and structure of proteins, materials and organisms [1] , [2] , [3] , [4] , in devices that exploit spin-dependent electron transport in solids (spintronics) [5] , [6] , in neutron scattering for structural characterization [7] , [8] and in quantum information experiments for preparation of pure initial states [9] , [10] . Dynamic nuclear polarization (DNP), in particular, comprises a family of techniques that transfer the greater spin polarization of electrons to nearby nuclei through hyperfine-mediated processes [11] , [12] . In a typical DNP experiment at high magnetic fields, stable paramagnetic centres (usually organic radicals) are introduced into an otherwise diamagnetic sample as a polarization source. The equilibrium polarization of electrons is sufficient to act as a polarization source for nuclei, because the gyromagnetic ratio of electrons is at least three orders of magnitude higher than that of nuclear spins [13] , [14] , [15] . In addition to the high magnetic field, the experiment requires cryogenic temperatures to attenuate competing spin-lattice relaxation processes, and it relies upon strong microwave irradiation near the electron precession frequency to accomplish polarization transfer. In alternative incarnations of this experiment that have been less generally applied, the initial electron polarization is produced by an optical pumping cycle involving the spin-orbit coupling [16] in a suitable substrate; the subsequent nuclear polarization can be controlled by electrical current in certain semiconductors and at cryogenic temperatures [17] , [18] , [19] . The negatively charged nitrogen-vacancy (NV) centre in diamond has been exploited in many applications, including solid-state magnetometry [20] , [21] , [22] , bioimaging and in single-photon sources [23] . Among its unique properties, the NV centre ( Fig. 1a ) can be prepared in a near-perfect state of electron spin polarization by optical illumination. Unlike in semiconductors that exhibit optical nuclear polarization, the high magnetic purity of the lattice in which the NV defect is situated, and the correspondingly long spin-lattice relaxation times, means that this can be accomplished even at room temperature. This feature makes diamond a particularly attractive substrate for spintronic devices or as a general source of polarization for NMR experiments, in which spin order can be transferred from a hyperpolarized diamond lattice to external spins of interest [24] , [25] . The utility of the NV centre in either application would be enhanced by the precise and non-inductive control over the lattice nuclear polarization, as is possible electrically in certain semiconductors but not for insulating solids [26] . Further, strongly coupled and polarized nuclear spins may serve both as quantum bits in information processing experiments and as auxiliary quantum registers that enhance the fidelity of certain quantum algorithms [27] , [28] , [29] . 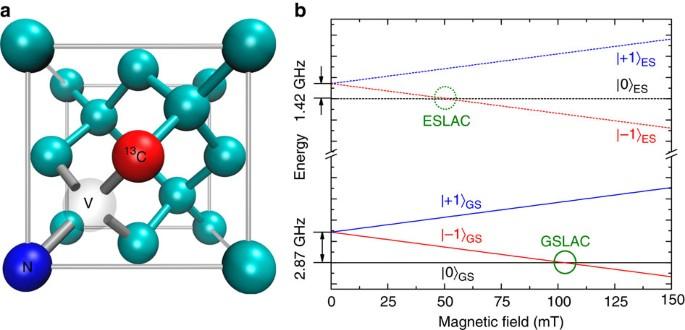Figure 1: Structure and energy diagram of NV in diamond. (a) Atomic representation of NV centre in diamond lattice with one of the first-shell carbon sites (Ca) occupied by13C (red). (b) The energy diagram of the ground-state triplet (3A, solid lines) and the excited-state triplet (3E, dashed lines) versus the magnetic field. The level anti-crossing occurs at ~51 mT in the excited state (ESLAC, dashed circle) and at ~102.5 mT in the ground state (GSLAC, solid circle). Figure 1: Structure and energy diagram of NV in diamond. ( a ) Atomic representation of NV centre in diamond lattice with one of the first-shell carbon sites (C a ) occupied by 13 C (red). ( b ) The energy diagram of the ground-state triplet ( 3 A , solid lines) and the excited-state triplet ( 3 E , dashed lines) versus the magnetic field. The level anti-crossing occurs at ~51 mT in the excited state (ESLAC, dashed circle) and at ~102.5 mT in the ground state (GSLAC, solid circle). Full size image The initial electron polarization of the NV results from optical pumping: the laser preferentially pumps the electron spin to the sublevel of the spin triplet ( 3 A ) ground state and creates electron spin polarization on the order of unity. This occurs because the electron spin goes through a spin-dependent intersystem crossing from the excited triplet state ( 3 E ), leading to enhanced spin polarization of the sublevel in the ground state [30] , [31] . The laser can be gated to switch the electron polarization on and off, but the polarization does not depend linearly on the laser intensity. In general, the electronic polarization of the NV centre is not accompanied by nuclear polarization because of the mismatch in the electron and nuclear resonance frequencies. However, the electrons and nuclei can exchange polarization if the hyperfine interactions have a non-negligible role in the dynamics of the system [24] . Such a condition can be established near the level anti-crossing in the excited state (ESLAC at ~51 mT, Fig. 1b ); near 100% polarization has been observed for nuclei such as 14 N or 15 N adjacent to the vacancy (that is, the nuclei of the nitrogen component of the NV centre), as well as proximal 13 C. In these experiments, the broad dependence of 14 N or 15 N polarization on magnetic field suggests the involvement of the isotropic component of the hyperfine interaction (the hyperfine interaction with 15 N or 14 N is isotropic in the excited state [32] , [33] ). The 13 C hyperfine couplings, on the other hand, are generally anisotropic in the ground state, and they vary with the lattice site [34] , [35] . As we will demonstrate below, the anisotropic hyperfine interaction can lead to a sharp dependence of electron-nuclear mixing, and hence nuclear spin polarization, on the magnetic field. This has been obscured in previous studies by the short lifetime of the excited state, and by the minimal electron-nuclear mixing in the ground state near the ESLAC condition due to the different zero-field splitting in the ground and excited states [24] , [25] . A level anti-crossing condition can also be reached in the ground state (GSLAC, or LAC for short, at ~102.5 mT, Fig. 1b ) [36] , whose long lifetime allows the electron-nuclear mixing to be probed in detail. Here, we demonstrate a near total nuclear polarization of an ensemble of the first-shell 13 C ( 13 C a , Fig. 1a ) coupled to NV near LAC. It is convenient to study 13 C a , because the strong hyperfine interaction allows the transitions associated with the NV- 13 C a pair to be clearly resolved from those of NV centres without 13 C a . We further investigated, experimentally and theoretically, the dependence of such nuclear polarization on the magnetic field. Probed by RF excitation in continuous-wave optically detected magnetic resonance (ODMR) spectra, the frequency distribution and the relative intensities of observed transitions reveal only one level anti-crossing condition for the NV- 13 C a pair, at a magnetic field slightly higher than that for NV without 13 C a . Near such level anti-crossing condition, the nuclear polarization depends sensitively on the magnetic field: at the most sensitive region near 105 mT, the nuclear polarization changes from ‘spin-up’ to ‘spin-down’ and back to ‘spin-up,’ within a few mT. The 13 C a spin polarization serves as an illustrative example for 13 C at other lattice sites with different hyperfine parameters. Indeed, the polarization and control mechanism should apply to all hyperfine-coupled 13 C, although each set of hyperfine parameters will give rise to a different nuclear polarization at the same magnetic field. ODMR spectra At a given magnetic field, the degree of electron-nuclear spin state mixing is determined by the energy separation between the electron and nuclear eigenstates and the relative contribution of the hyperfine interaction to the total Hamiltonian (that is, the matrix elements connecting these states). This also determines the energy levels and the resulting transition frequencies between the two mixed states that are eigenstates of the perturbed Hamiltonian. In turn, the intensities of the various transitions depend on the populations of the mixed states, and both the frequencies and the relative intensities of allowed transitions can be measured in ODMR spectra [24] . 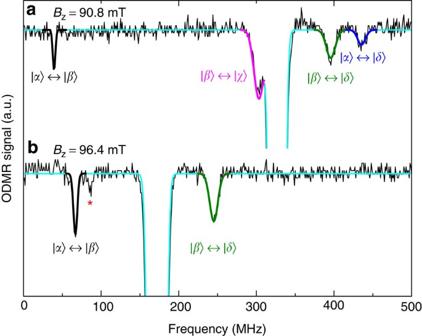Figure 2: Representative ODMR spectra near LAC. The spectra are acquired at (a)Bz=90.8 mT with four peaks associated with NV-13Capairs clearly resolved, and (b)Bz=96.4 mT, above which thetransitions disappear. The spectra are averaged over 2,000 scans. All peaks are fit to Gaussian lineshapes. The intense primary peak associated with NV centres without13Cais used to determine the magnetic field as shown in light blue solid lines. The weaker peaks associated with NV-13Capairs are colour-coded and labelled according to the related transitions determined inFig. 4a. The peak labelled by a red * is an artefact whose second harmonic matches the frequency of the main peak. Figure 2 shows representative ODMR spectra of the NV ensemble near LAC (see Supplementary Figs S1, S2 for spectra at ambient magnetic field and near LAC, respectively). The smaller peaks that are resolved from the intense primary peak are assigned to NV centres coupled to 13 C a (refs 33 , 35 , 37 ). As there are only three equivalent C a sites for each NV, and because of the low natural abundance of 13 C (1.1%), the peak intensities (that is, integrated area of the peak) associated with NV- 13 C a pairs are much smaller than the primary peaks originating from the greater fraction of NV centres without 13 C a . The spectra taken near LAC may have one, two, three or four peaks, and are thus different from the spectra taken at ambient or low (<10 mT) magnetic field, where the two peaks associated with NV- 13 C a pairs are separated by ~130 MHz and asymmetrically located on either side of the primary peaks [37] . The number of observed resonances near LAC suggests that the electron-nuclear spins are in mixed states. Were this not the case, the selection rules permit only two electron spin transitions to be observed optically, each of which is associated with one nuclear spin state [28] . Figure 2: Representative ODMR spectra near LAC. The spectra are acquired at ( a ) B z =90.8 mT with four peaks associated with NV- 13 C a pairs clearly resolved, and ( b ) B z =96.4 mT, above which the transitions disappear. The spectra are averaged over 2,000 scans. All peaks are fit to Gaussian lineshapes. The intense primary peak associated with NV centres without 13 C a is used to determine the magnetic field as shown in light blue solid lines. The weaker peaks associated with NV- 13 C a pairs are colour-coded and labelled according to the related transitions determined in Fig. 4a . The peak labelled by a red * is an artefact whose second harmonic matches the frequency of the main peak. Full size image Theoretical calculations of energy levels and eigenstates The relevant NV spin Hamiltonian, including its hyperfine interaction with 13 C a , is given by [38] , [39] , [40] : where the axial ( D =2,870 MHz) and transverse ( E , a strain splitting particular to each diamond sample; for our sample, E =3.5 MHz) zero-field splitting parameters are determined from the spectra at ambient magnetic field (see Supplementary Fig. S1 ), S is the electron spin of NV with the electron gyromagnetic ratio of γ e , z is defined along the NV symmetry axis, B is the external magnetic field, I is the 13 C a nuclear spin with the gyromagnetic ratio , and A is the hyperfine-interaction tensor between NV and 13 C a , given by A ┴ =123 MHz and A ‖ =205 MHz, with its principal axis ~74° relative to the symmetry axis of the NV as characterized by ESR [41] . This hyperfine tensor can also be quantized along the NV symmetry axis through a rotation [12] , [42] : where the x axis lies within the NV- 13 C a plane, and y is perpendicular to the NV- 13 C a plane, forming orthogonal coordinates ( Supplementary Fig. S3 ), and the ladder operators are S ± = S x ± i · S y and I ± = I x ± i · I y . The Hamiltonian can then be diagonalized near LAC to obtain the energy levels ( Fig. 3a ) and eigenstates ( Fig. 3b and Supplementary Figs S4, S5 ). The mixed states, namely , , and , are defined as in Fig. 3a . Near the LAC, the energy of the and sublevels converge, and all terms in Equation (2) contribute to the dynamics and cannot be truncated [12] , [42] . The off-diagonal hyperfine elements may give rise to additional level anti-crossing conditions and provide a polarization transfer mechanism via simultaneous electron-nuclear flip-flops. For instance, the crossings of the eigenstate projections in Fig. 3b correspond to level anti-crossing conditions [37] , [39] , among which is the near-crossing between and at ~100 mT (LAC−) and the crossing between and at ~105 mT (LAC+). They are caused by the S − I + and S − I − hyperfine elements, respectively, near LAC at ~102.5 mT. 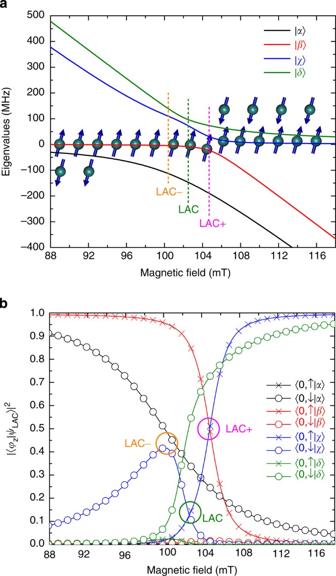Figure 3: Theoretical calculations of energy levels and eigenstates of the NV-13Casystem. (a) Energies of the four eigenstates near LAC. The LAC−, LAC and LAC+ are labelled by vertical dashed lines. The spin symbols illustrate how the polarization evolves at different magnetic field strengths, given the dominant nuclear projection of each state. (b) Eigenstates are expressed by their projections onto thestates of the NV-13Capair, whereandare electron and nuclear quantum numbers, respectively. The LAC−, LAC, and LAC+ are labelled by circles. Figure 3: Theoretical calculations of energy levels and eigenstates of the NV- 13 C a system. ( a ) Energies of the four eigenstates near LAC. The LAC−, LAC and LAC+ are labelled by vertical dashed lines. The spin symbols illustrate how the polarization evolves at different magnetic field strengths, given the dominant nuclear projection of each state. ( b ) Eigenstates are expressed by their projections onto the states of the NV- 13 C a pair, where and are electron and nuclear quantum numbers, respectively. The LAC−, LAC, and LAC+ are labelled by circles. Full size image The observed level anti-crossing condition The NV electron spin is polarized to the state under laser irradiation [43] , [44] . However, it is unclear how the spin population is distributed among the four electron-nuclear mixed states when the two electronic states are split by the large hyperfine interaction near LAC. Resolved ODMR spectra might provide such detailed information, if each observed peak can be assigned to a pair of eigenstates connected by the transition. 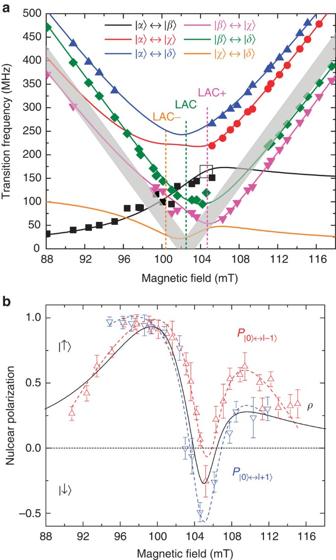Figure 4: Transition assignments for the estimation of nuclear polarization. (a) Assignment of the observed transitions (solid symbols) based on frequency in comparison with theoretical calculation (solid lines). Some allowed transitions related to the NV-13Capair may be obscured by the main peak from NV without13Ca(grey area with its width determined by the intense primary peak). The region where certain transitions near LAC+ disappear is shown by an open black square. (b) Nuclear polarization measured via different electronic sublevels of the NV.is shown in red up triangles,(with artefacts from the solid effect removed) is shown in blue down triangles. The black line is the calculated spin flip-flop probability (ρ) resulting from the combined effect of theS−I+andS−I−hyperfine elements. The red and blue dashed lines are fitting curves based on two Lorentzian functions forand, respectively, that resemble the features ofρ. The error bars are propagated from the s.e. of the parameters used for Gaussian fittings of peaks in the ODMR spectra, and the subsequent area integration of each individual peak. Figure 4a shows a comparison of the observed transition frequencies with those calculated from the energy levels as shown in Fig. 3a . The excellent agreement confirms that the low-intensity peaks originate from the NV- 13 C a pairs and enables each observed transition to be unambiguously assigned to a pair of eigenstates. Figure 4: Transition assignments for the estimation of nuclear polarization. ( a ) Assignment of the observed transitions (solid symbols) based on frequency in comparison with theoretical calculation (solid lines). Some allowed transitions related to the NV- 13 C a pair may be obscured by the main peak from NV without 13 C a (grey area with its width determined by the intense primary peak). The region where certain transitions near LAC+ disappear is shown by an open black square. ( b ) Nuclear polarization measured via different electronic sublevels of the NV. is shown in red up triangles, (with artefacts from the solid effect removed) is shown in blue down triangles. The black line is the calculated spin flip-flop probability ( ρ ) resulting from the combined effect of the S − I + and S − I − hyperfine elements. The red and blue dashed lines are fitting curves based on two Lorentzian functions for and , respectively, that resemble the features of ρ . The error bars are propagated from the s.e. of the parameters used for Gaussian fittings of peaks in the ODMR spectra, and the subsequent area integration of each individual peak. Full size image Based on the distribution of the observed transitions over an ~30 mT range near LAC, only one level anti-crossing condition is observed for NV- 13 C a pairs, at LAC+, even though each off-diagonal hyperfine element, in principle, introduces an additional level anti-crossing condition. The first signature of this condition is the discontinuous disappearance of the transition and the appearance of the and transitions as B z crosses LAC+ ( Fig. 4 ). Absent the hyperfine interaction, the transition frequency changes continuously as the energy of the polarized state becomes greater than that of the state, when B z crosses the LAC ( Fig. 1b ). This was previously identified by the inverted phase of the ESR signal when sweeping the magnetic field across LAC [45] . Further, due to the anisotropic hyperfine interaction we anticipate a frequency change when the polarized state goes from the lower to higher energy levels at the level anti-crossing condition, which is exactly what we observed at LAC+ ( Fig. 4a ). The second signature is the disappearance of the transition between 104 mT and 105 mT (within the open black square in Fig. 4 ), because the population in the state becomes small, which was also shown by ESR [45] . Similar phenomena are not observed at LAC−. These observations suggest that the mixed state with the greatest polarization or population changes from to at LAC+, but not from to at LAC−. These phenomena follow from the form of the anisotropic hyperfine Hamiltonian responsible for electron-nuclear polarization transfer. The NV electron spins are optically pumped to the sublevel, but as the and sublevels approach degeneracy near LAC, the only available electronic transitions for the transfer of polarization are the S − I + or S − I − hyperfine elements. As the S − I + hyperfine element has much larger magnitude than that of S − I − in Equation (2), the former effectively pumps the nuclear spin to the state over a wide range of magnetic fields (with an exception discussed in the following section). The combined effect of continuous laser irradiation and polarization transfer therefore tends to populate the state. This explains why only LAC+ is observed, occurring at the magnetic field where the two mixed states with the largest component, namely and , meet the level anti-crossing condition ( Fig. 3b ). The polarization of the electron-nuclear mixed states With each transition assigned to the mixed states and the effective level anti-crossing conditions identified, the relative peak intensities within the same spectrum reveal the spin polarization below and above LAC+. The spin polarization among the four mixed states is illustrated in Fig. 3a and can be explained as follows: from ~88 to ~105 mT, (the integrated area of the peak) decreases until it completely disappears above ~96 mT, while continues to increase up to ~105 mT ( Fig. 2 ). This suggests that the spin population of is gradually pumped into , with nearly complete polarization in the state above ~96 mT ( Fig. 2b and Supplementary Fig. S2a ). This occurs as the combined effect of optical pumping and the hyperfine element near LAC− tends to pump the spins to , which is the primary component of the state below ~105 mT ( Fig. 3b ). The same effect also suggests that is the most polarized state above ~106 mT, where has the largest projection onto . This is indeed observed, as demonstrated by the larger intensity of and compared with that of ( Supplementary Fig. S2c ). The level anti-crossing at LAC+ thus changes the most polarized state from to . However, within a narrow range of 105–106 mT near LAC+, is observed to be smaller than ( Supplementary Fig. S2b ), suggesting that the spin population in is slightly larger than that in . This occurs as has its largest projection onto within this field range, so the optical pumping mechanism tends to preferentially populate ( Fig. 3b ). As the major projection component of the state at LAC+ is ( Fig. 3b ), the S − I − hyperfine element, instead of S − I + , must dominate the polarization transfer processes. The competing effect between S − I + and S − I − hyperfine elements will be further discussed in the following section. Our tabulation of observed transition frequencies demonstrates how spin polarization is affected by the anisotropic hyperfine interaction near the level anti-crossing. The detailed observation of spin polarization and its dependence on the magnetic field provide insights into the mechanism of electron and nuclear spin polarization using the NV centre [43] . Nuclear polarization and its dependence on magnetic field Both the polarization of the electron-nuclear mixed states and their projections onto each nuclear spin state depend on the magnetic field, suggesting that the nuclear polarization should as well. In addition to the eigenstates we have calculated ( Fig. 3b and Supplementary Figs S4, S5 ), we must know the spin population of each electron-nuclear mixed state in order to determine the nuclear polarization. In principle, the spin population can be calculated from the peak intensities of all transitions between any two mixed states (out of six transitions in total). However, not all transitions associated with NV- 13 C a pairs can be individually resolved; several transitions are obscured by the large peak arising from NV centres that are not coupled to 13 C a (the grey area in Fig. 4a ). In order to estimate the nuclear polarization, we assume that the ratio of the intensities of two individual peaks, such as and , approximates the ratio of spin populations in the and states, respectively, (see Methods for the estimation of nuclear polarization). We further assume that the electron spin polarization is near unity. The estimated nuclear polarization measured via the transition ( , red up triangles) is shown in Fig. 4b as a function of the magnetic field. The nuclear polarization increases as B z increases until ~96 mT, because the normalized spin population in ( p β ) is much greater than that of ( p α ), leading to almost complete nuclear polarization. Such polarization decreases to zero and changes sign near LAC+. Above LAC+, the spin distribution among and causes the polarization to increase up to 60% before decreasing to 30% at ~115 mT. In order to obtain a complete picture of the spin dynamics and an independent estimate of the nuclear polarization, we also measured the ODMR spectra via the transition. The frequencies and assignments of observed transitions are shown in Supplementary Fig. S6 . These results largely agree with those accomplished by measurement via the transitions. For example, the signatures of level anti-crossing conditions are also observed at LAC+. The polarization of the electron-nuclear mixed states agrees with the measurement via the transitions ( Fig. 3a ): from ~94 to ~103 mT, all observed transitions are associated with the state; within a narrow range near LAC+, is the most polarized mixed state; and all transitions are associated with either or above LAC+. Our observations of the transition ( Supplementary Fig. S6 ), however, indicate that there is an additional nuclear polarization mechanism induced by the applied microwave field. Specifically, the transition is usually forbidden under the selection rules. In the presence of hyperfine interaction, the eigenstates in the manifold are no longer pure states near LAC (for instance, , in Fig. 3b ). A resonant microwave field can excite transitions from this manifold of eigenstates that are mixed basis states to the sublevels. These transitions are forbidden in the basis of pure states (that is, simultaneous flip-flop of the electron and nuclear spins). This mechanism of dynamic nuclear polarization is the well-known solid effect, documented in the literature [11] , [12] , [46] and routinely employed for sensitivity enhancement in paramagnetically doped solids. Under our experimental conditions, we estimate that the nuclear polarization at 94.9 mT is only ~43% when the solid effect is considered, as compared with ~100% without the solid effect ( Supplementary Fig. S7 ). As the solid effect operates only at a narrow resonance condition (a given microwave frequency at a given magnetic field), only the seemingly forbidden transition ( ), is affected. The rest of the observed peaks (all other transitions but in Supplementary Fig. S6 ) are associated with allowed transitions that can be used to estimate the nuclear polarization with artefacts from the solid effect removed ( , blue down triangles in Fig. 4b , see Methods). We thus use only these in our calculations. Under the condition such that the hyperfine interaction causes strong electron-nuclear spin mixing between the and sublevels near LAC, the dynamics within this manifold are explained largely by allowed, rather than forbidden, transitions; thus the solid effect does not contribute to the polarization measured via the transition. The observed nuclear polarization can be explained by the probability of the electron-nuclear spin flip-flop induced by the S − I + ( ρ ↑ ) and S − I − ( ρ ↓ ) hyperfine elements [24] . The transition probabilities corresponding to each hyperfine element can be calculated from the degree of mixing between relevant eigenstates [24] (see Methods and Supplementary Fig. S8 ). It is clear that is relatively larger over the entire range of magnetic field in this study (88–118 mT) except the region of 104–106 mT where ρ ↓ is larger. The combined effect ( ρ , black line in Fig. 4b ) explains the pattern of nuclear polarization as a function of magnetic field. Both experimentally measured estimates for the nuclear polarization, and , agree with the predicted to a good approximation. The seems to be more accurate than , because the former estimate is based on transitions from a mixed state to a nearly pure state and all transitions are resolved, whereas the latter is based on transitions between two mixed states and not all transitions can be resolved. For instance, tends to overestimate the nuclear polarization within the magnetic field of 102–112 mT. Nevertheless, both measurements show a nearly complete nuclear polarization near LAC− and inverted polarization to nuclear spin down at LAC+, confirming the sensitive dependence on the magnetic field and the assumptions of our theory. As we have demonstrated elsewhere [47] , shaped optical irradiation can be used to produce a time- and space-varying pattern of polarization up to the diffraction limit; here we demonstrate that the magnetic field can act as a complementary control parameter. The anisotropic hyperfine interaction of NV centres with the surrounding lattice carbons in diamond allows the magnetic field to be used as an active and sensitive control of the nuclear polarization near 105 mT (LAC+). The effect of the hyperfine interaction is pronounced only at the near-degeneracy condition of electronic states, which is at the level anti-crossing for the NV centres in diamond. A similar nuclear polarization mechanism has also been used in GaAs semiconductors at the fractional quantum Hall regime with a filling factor of v =2/3 (refs 48 , 49 , 50 ). When the cyclotron energies of the first two Landau levels match the electron spin Zeeman energy at the filling factor of v =2/3, the electronic states become nearly degenerate and the nuclear spin can be polarized by electrical current and measured by resistivity [50] . Unfortunately, cryogenic temperatures (<4.2 K) and high magnetic field (a few tesla) are generally required for such nuclear polarization in semiconductors. The advantages of the NV centre in diamond, by contrast, are that similar control over polarization can be achieved at room temperature and low magnetic field (~0.1 T). The combination of optical pumping and initialization, precise magnetic control and optically detected polarization as demonstrated here are a complete set of non-inductive techniques that are potentially useful for nuclear-based spintronics in insulating or semiconducting diamonds [23] , [26] . Our experiments, demonstrating complete polarization of the 13 C nuclei at ~0.1 T and room temperature, together with the results of King et al. [51] demonstrating transport of polarization to bulk nuclei via spin diffusion at ~9.4 T, suggest that the bulk polarization of 13 C nuclei in our diamond sample approaches several per cent [52] . Thus, our method may be applied wherever hyperpolarized bulk 13 C nuclei are required [51] , including in DNP-enhanced NMR experiments, in spintronic devices and for NV-based devices including magnetometers and gyroscopes [53] . Materials and experiments The diamond used in our experiments (labelled S9 in previous studies [22] , [54] ) contains ~2 p.p.m. of negatively charged NV. A continuous beam from a 532-nm laser with optical power of 2 mW is focused on the diamond by an objective with a numerical aperture of 0.7 to achieve optical power density of ~5 mW μm −2 . The fluorescence signal from NV is detected by an avalanche photo detector after passing a dichroic mirror and a long-pass filter [54] . The external magnetic field is applied with a permanent magnet aligned to one of the NV symmetry axes with a precision better than ~1°, otherwise the large transverse magnetic field may obscure the effect of the off-diagonal hyperfine elements. The strength of the magnetic field is adjusted by the distance of the magnet from the laser focus point on the diamond. The magnetic field is determined precisely using the NV without proximal 13 C a nuclei acting as a magnetometer; the central frequencies of the intense primary peaks in the ODMR spectra are directly related to the magnetic field [22] . A single copper wire loop arranged about the laser focus produces an oscillating RF magnetic field with Rabi frequency ~350 kHz. The ODMR spectra are measured by recording the fluorescence intensity while the excitation frequency is scanned from 1 to 500 MHz for the transition (or from 5.4 to 6.1 GHz for the transition) and are normalized to the fluorescence intensity obtained without RF excitation. Estimation of nuclear polarization Assuming that the electron polarization is near 100%, almost all spin population resides either at or at below LAC+, and either at or at above LAC+, that is, the normalized spin population ( ) is approximately given by p α + p β =1 and p χ = p δ =0 below LAC+. In addition, the ODMR peak intensity is also affected by the optical contrast between and . Below LAC+, the spin population can be related to the observed peak intensities of and by considering the fluorescence contrast of the two states: The nuclear polarization measured via the transition, , can be estimated based on the polarization among the mixed states and their projections onto each nuclear spin state: The transitions associated with are obscured by the main peak (the grey area in Fig. 4a ), and we may disregard these transitions under the assumption that p χ = p δ =0. A similar method is used to calculate above LAC+ by comparing with , and by assuming that p α = p β =0 and p χ + p δ =1. Here, is used instead of , because the and transitions approach the same frequency (the two peaks merge) as the magnetic field increases above ~118 mT. The comparison between and therefore more accurately represents the nuclear polarization above LAC+. The nuclear polarization measured via the transition with artefacts from the solid effect removed, , is estimated by first comparing the intensities of the transitions to ( ) and to ( ) in the ODMR spectra other than the forbidden transition due to the solid effect ( ), for instance via, The projections onto each nuclear spin state is then included via, A similar method is used to calculate below LAC+ by using and also for the magnetic field within 102–105 mT. Probability of electron-nuclear spin flip-flop The probability of electron-nuclear spin transitions induced by the S − I + ( ρ ↑ ) and S − I − ( ρ ↓ ) hyperfine elements are calculated by the degree of mixing between relevant eigenstates shown in Fig. 3b (ref 24 ): where both and for ρ ↑ are considered because of the mixing effect due to S z I x . The calculated probabilities and their combined effect ( ρ = ρ ↑ −ρ ↓ ) are shown in Supplementary Fig. S8 . How to cite this article: Wang, H. -J. et al. Sensitive magnetic control of ensemble nuclear spin hyperpolarization in diamond. Nat. Commun. 4:1940 doi: 10.1038/ncomms2930 (2013).